Transport spectroscopy of non-equilibrium many-particle spin states in self-assembled quantum dots Self-assembled quantum dots (QDs) are prominent candidates for solid-state quantum information processing. For these systems, great progress has been made in addressing spin states by optical means. In this study, we introduce an all-electrical measurement technique to prepare and detect non-equilibrium many-particle spin states in an ensemble of self-assembled QDs at liquid helium temperature. The excitation spectra of the one- (QD hydrogen), two- (QD helium) and three- (QD lithium) electron configuration are shown and compared with calculations using the exact diagonalization method. An exchange splitting of 10 meV between the excited triplet and singlet spin states is observed in the QD helium spectrum. These experiments are a starting point for an all-electrical control of electron spin states in self-assembled QDs above liquid helium temperature. Epitaxial semiconductor quantum dots (QDs) are nanoscale objects, which incorporate fully confined carriers and are therefore perfectly suited for fundamental studies on atom-like objects in a solid-state environment [1] , [2] . In addition, these structures are promising building blocks for future quantum information processing [3] , [4] . These visionary applications require a controlled preparation of non-equilibrium states with well-defined charge and spin degrees of freedom. For self-assembled QDs, great progress has been made in this field using optical excitation and detection methods [5] , [6] , [7] , [8] , [9] , [10] , [11] . Optical techniques, however, may be difficult to implement in highly integrated (classical or quantum) computer technologies. An all-electrical preparation and time-resolved detection of non-equilibrium QD states are therefore highly desirable, but have so far only been achieved in lithographically defined QDs [12] , [13] , [14] , [15] at very low temperatures (mK). In this study, we use a novel all-electrical measurement technique to prepare and detect the ground and excited many-particle spin states in self-assembled InAs QDs at liquid helium temperature. This way, the pure electron spectra of QD hydrogen, helium and lithium are resolved. Comparison with detailed many-particle calculations enables us to identify the different charge and spin configurations in the spectra and in particular to detect the singlet and triplet states of QD helium. Furthermore, the possibility for time-resolved measurements is demonstrated and the evolution from non-equilibrium to equilibrium occupation is investigated. This constitutes an important step towards electrical quantum operations in self-assembled QDs. 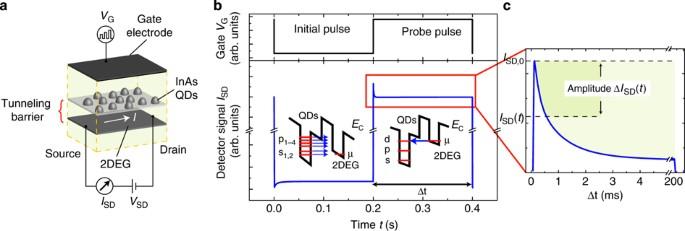Figure 1: Schematic sample geometry and measurement technique. (a) The transistor structure, which is used to record the time-dependent tunnelling into self-assembled QDs. A voltage pulse applied to the gate electrode (b) (top) will abruptly change the carrier density in the electron channel (2DEG). The corresponding change in resistance is observed in the time-resolved measurement of the source-drain currentISD(VSD= constant) (b) (bottom). The voltage pulse will also strongly shift the chemical potential of the dots embedded in the dielectric between the gate and the 2DEG. This creates a non-equilibrium situation, in which electrons from the 2DEG can tunnel into excited QD states (right inset) (b). The time-dependent transfer of charge into the dots,QQD(t), will cause a decrease in carrier density of the 2DEG, which is detected by recording the change in source-drain current ΔISD(t) (c). Time-resolved conductance spectroscopy The investigated sample consists of an inverted high electron mobility transistor (HEMT) with an embedded ensemble of self-assembled InAs QDs [1] , [16] , [5] ; see Figure 1a and the Methods section for details. As the electron channel, which supplies the carriers for the QDs, we employ a two-dimensional electron gas (2DEG) [17] . The tunnelling barrier between the 2DEG and QDs was chosen so that the tunnelling time is in the range of a few milliseconds. When a voltage pulse is applied to the gate, the carrier density and thus the conductivity of the 2DEG will change with a short RC time constant t RC =300 μs. At the same time, the energy levels of the dots, embedded in the dielectric of the HEMT, will shift [1] and electrons will start to tunnel between the 2DEG and the dots. This increase in the number of electrons per dots will lead to a time-dependent decrease of the carrier density in the 2DEG [18] , which can be monitored with a high resolution by recording its conductivity. Thus, applying a constant voltage across the source and drain of the HEMT and recording the current transient I SD ( t ) will give a direct measure of the time-dependent tunnelling into the dots [19] . Because the response time of the 2DEG to an applied gate voltage pulse is much shorter than the typical tunnelling times, the present setup allows us to prepare non-equilibrium situations, in which the chemical potentials in the 2DEG and the dot layer differ greatly and tunnelling can take place over a wide range of energies (see insets in Fig. 1b ). As we will show in the following section, this makes it possible to investigate excited QD states, as in n − i − n tunnelling structures [20] , [21] , however, with adjustable, well-defined initial charge (zero, one or two electrons per dot). Figure 1: Schematic sample geometry and measurement technique. ( a ) The transistor structure, which is used to record the time-dependent tunnelling into self-assembled QDs. A voltage pulse applied to the gate electrode ( b ) (top) will abruptly change the carrier density in the electron channel (2DEG). The corresponding change in resistance is observed in the time-resolved measurement of the source-drain current I SD ( V SD = constant) ( b ) (bottom). The voltage pulse will also strongly shift the chemical potential of the dots embedded in the dielectric between the gate and the 2DEG. This creates a non-equilibrium situation, in which electrons from the 2DEG can tunnel into excited QD states (right inset) ( b ). The time-dependent transfer of charge into the dots, Q QD ( t ), will cause a decrease in carrier density of the 2DEG, which is detected by recording the change in source-drain current Δ I SD ( t ) ( c ). Full size image Figure 1b shows the measurement procedure. First, a well-defined QD state is prepared by setting an initial bias V ini and giving the system enough time (0.1 s) to equilibrate. Then, the probe pulse V p is applied and I SD is recorded as a function of time ( Fig. 1c ). For better signal-to-noise ratio, I SD ( t ) is averaged over 1,000 pulses. As mentioned above, I SD ( t ) is proportional to Q QD . Therefore, in equilibrium ( t →∞) its derivative with respect to the gate voltage dΔ I SD /d V p is proportional to the (quantum) capacitance of the layer system, which is given by the density of states in the QDs [17] . The non-equilibrium situation is more complex; however, model calculations (not shown here) and experiments by Vdovin et al . [20] show that also in non-equilibrium, the derivative of the tunnelling current amplitude versus the gate voltage reflects the density of states. Therefore, by plotting dΔ I SD /d V p , the complete time evolution of the QD states can be obtained as the dots are filling up with electrons. Gate voltages V p can be converted to energies using the well-established lever arm model Δ E = e Δ V p /λ, where the lever arm λ= d gate / d QD=6 is given by the distance d QD between 2DEG and dots and the distance d gate between 2DEG and gate. 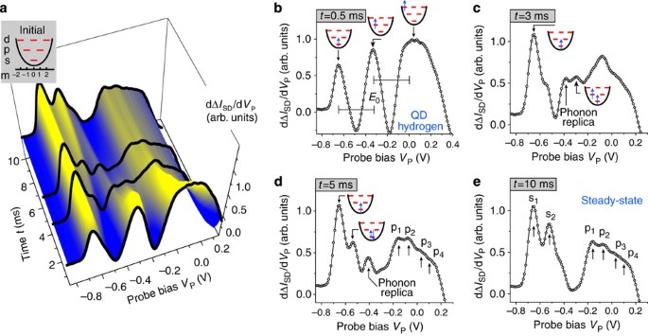Figure 2: Time evolution of the QD charging spectrum. (a) Coloured surface plot of dΔISD/dVp—corresponding to the QD states—as a function of time and pulse biasVp. The initial bias is set so that the QDs are empty att=0. The inset in (a) illustrates the harmonic model potential, together with the common labels for the QD states and their angular momentumm. (b–e) show the charging spectra for different time delays. The electron configurations of the final states, obtained from a comparison between measured and calculated energies, is depicted above the different resonances. For the shortest possible time delay of 0.5 ms (b), the data exhibit roughly equidistant charging peaks, as expected from the single-particle harmonic oscillator model. At aroundt=3 ms (c), many-particle charging peaks start to appear, and tunnelling into the ground and excited states of the two-electron system ('QD helium') is visible atVp=−0.53 V andVp=−0.26 V, respectively. An additional structure atVp=−0.4 V (d) is caused by a phonon replica of the lowest single-electron charging process. Att=10 ms (e), the system is close to equilibrium and the charging peaks resemble those found in capacitance spectroscopy, with two s-states (s1and s2separated by the Coulomb energy) and a broad structure with the four p-states. Time-evolution of the spectrum Figure 2a displays a three-dimensional plot of dΔ I SD /d V p spectra for a transient time t between 0.5 ms and 10 ms. The initial bias is set to V ini =−0.9 V, so that the dots are completely empty before V p is applied. The data demonstrates how the QD states in the ensemble evolves, as the dots are filled subsequently with up to six electrons. Figure 2: Time evolution of the QD charging spectrum. ( a ) Coloured surface plot of dΔ I SD /d V p —corresponding to the QD states—as a function of time and pulse bias V p . The initial bias is set so that the QDs are empty at t =0. The inset in ( a ) illustrates the harmonic model potential, together with the common labels for the QD states and their angular momentum m . ( b – e ) show the charging spectra for different time delays. The electron configurations of the final states, obtained from a comparison between measured and calculated energies, is depicted above the different resonances. For the shortest possible time delay of 0.5 ms ( b ), the data exhibit roughly equidistant charging peaks, as expected from the single-particle harmonic oscillator model. At around t =3 ms ( c ), many-particle charging peaks start to appear, and tunnelling into the ground and excited states of the two-electron system ('QD helium') is visible at V p =−0.53 V and V p =−0.26 V, respectively. An additional structure at V p =−0.4 V ( d ) is caused by a phonon replica of the lowest single-electron charging process. At t =10 ms ( e ), the system is close to equilibrium and the charging peaks resemble those found in capacitance spectroscopy, with two s-states (s 1 and s 2 separated by the Coulomb energy) and a broad structure with the four p-states. Full size image Let us first consider the spectra for the shortest possible time delay t =0.5 ms≥ t RC . In the present structure, the tunnelling times between the 2DEG and the dots are in the order of τ s =6 ms and τ p =1.4 ms for the s- and p-states, respectively [18] , so that at t =0.5 ms, to a good approximation, only tunnelling from the empty to the singly occupied dots is observed. As shown in Figure 2b , we observe three equidistant peaks in the signal, with a spacing of 52 meV, which is in good agreement with previous studies [16] . However, this measurement shows for the first time degenerate electron states without Coulomb interaction. The final state configuration of the tunnelling process is sketched above each peak: at V p =−0.65 V, electrons resonantly tunnel into the lowest (s-) state of the dots; at V p =−0.34 V, non-equilibrium tunnelling into the degenerate p-states takes place; and at around V p =0.05 V, electrons are injected directly into the d-shell. Figure 2c,d shows the spectra for intermediate delay times t ≈τ s, τ p . Features from tunnelling into both equilibrium and non-equilibrium states can be observed. For example, the spectrum at t =3 ms exhibits peaks at both V p =−0.53 V (more clearly seen in Fig. 2d ) and −0.29 V. Comparison with theory (see below) allows us to identify these resonances as tunnelling into the ground and excited state of the doubly occupied dot (QD helium). Also, a new resonance at −0.4 V appears, which cannot be explained by an equilibrium or non-equilibrium state in the dots. From the fact that—compared with the lowest (s 1 ) resonance—it exhibits a constant energy difference of about 41 meV and a constant amplitude, we conclude that this resonance is a phonon replica [22] of the s 1 -state caused by efficient scattering of tunnelling electrons by inelastic LO phonons in the strained GaAs barrier [23] . In the opposite limit, t τ s ,τ p , the amplitude Δ I SD ( V p , t →∞) corresponds to the total charge in the dots under equilibrium conditions, and the signal dΔ I SD /d V p will reflect the equilibrium, many-particle spectrum of the dots. For the longest time delay shown here (10 ms), we find two maxima around V p =−0.6 V and a broad structure ranging from −0.24 V to +0.2 V. Comparison with the results from capacitance spectroscopy [17] shows that the first two resonances are the two s-states of the QDs, which are separated by ≈20 meV because of Coulomb interaction. The broad structure is a signature of the four resonances of the p-shell (see arrows in Fig. 2e ). QD elements Even though many features of equilibrium and non-equilibrium tunnelling can be identified in the time-resolved evolution shown in Figure 2 , the fact that signals from dots with different occupations are superimposed makes a detailed interpretation of these data difficult. Therefore, in the following section, we will ensure a well-defined tunnelling process n −1→ n by setting V ini so that n −1 electrons are present in the dots when the probe pulse is applied and that considering only the shortest possible time delay, so that higher-order tunnelling processes Δ n =2 are strongly suppressed. The number of electrons in the final state determines which QD 'element' is being investigated: QD hydrogen, helium or lithium for n =1, 2 and 3, respectively. QD hydrogen has already been discussed above (see Fig. 2b ). Here, the spectroscopy of the equidistant excited energy levels with a spacing of ħω =52 meV provides valuable input for the theoretical treatment of the many-particle states. 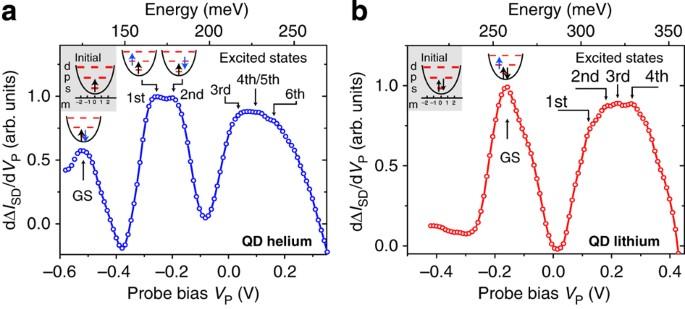Figure 3: Spectroscopy of excited states in QD helium and lithium. (a,b) Charging spectra for tunnelling into the two- and three-electron final states, respectively, taken at the shortest possible time delayt=0.5 ms. The initial states, prepared by appropriately settingVini, are depicted in the upper left corner of each panel. The electron configurations, drawn above the measured resonances, are taken from a comparison with theoretical calculations. For QD helium, we observe the lowest resonance atVp=−0.53 V caused by tunnelling into the two-electron ground state (GS) s2. Around −0.25 V, a double-peak structure is seen corresponding to tunnelling into the p-shell. The splitting is caused by the difference in exchange energy between the triplet (Vp=−0.26 V) and the singlet (Vp=−0.2 V) excited state. Three further resonances can be identified around +0.1 V, which are caused by tunnelling into the excited d-shell. For QD lithium, also a clear separation between tunnelling into ground and excited states is possible. Through comparison with the calculated spectrum, the fine structure can be identified as the first four excited states of the three-electron system. The spectrum of QD helium is shown in Figure 3a . We find a resonance at V p =−0.53 V, which can be identified as tunnelling into the two-electron ground state (GS; s 2 ), in agreement with equilibrium measurements [18] and the results in Figure 2 . Further resonances can be identified at V p =−0.26 V and −0.2 V as well as a broad peak around V p =+0.1 V. QD lithium is shown in Figure 3b , in which V ini =−0.44 V was chosen so that two electrons occupy the lowest (s) shell and the third electron can be injected either into the p- or the d-shell. One resonance is observed at −0.16 V and four further resonances between +0.06 V and +0.4 V. Figure 3: Spectroscopy of excited states in QD helium and lithium. ( a , b ) Charging spectra for tunnelling into the two- and three-electron final states, respectively, taken at the shortest possible time delay t =0.5 ms. The initial states, prepared by appropriately setting V ini , are depicted in the upper left corner of each panel. The electron configurations, drawn above the measured resonances, are taken from a comparison with theoretical calculations. For QD helium, we observe the lowest resonance at V p =−0.53 V caused by tunnelling into the two-electron ground state (GS) s 2 . Around −0.25 V, a double-peak structure is seen corresponding to tunnelling into the p-shell. The splitting is caused by the difference in exchange energy between the triplet ( V p =−0.26 V) and the singlet ( V p =−0.2 V) excited state. Three further resonances can be identified around +0.1 V, which are caused by tunnelling into the excited d-shell. For QD lithium, also a clear separation between tunnelling into ground and excited states is possible. Through comparison with the calculated spectrum, the fine structure can be identified as the first four excited states of the three-electron system. Full size image For a thorough identification of the different resonances, we have calculated the many-particle energy states in a 2D harmonic oscillator for n =1, 2 and 3 electrons using the exact diagonalization method, which provides numerically exact solutions [24] , [25] . This yields the many-particle states of the interacting electrons in terms of superpositions of single-particle Slater determinants. Their coefficients give the probability of single-particle configuration to be found. The level spacing ħω =52 meV was taken from the single-particle spectrum in Figure 2b . The effective mass and the dielectric constant were chosen to be m * =0.067 m 0 and ɛ r =16, respectively, which go into the calculations by the single adjustable parameter [16] . 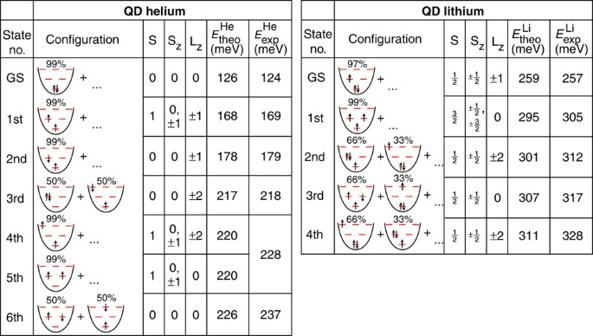Figure 4: Calculated excitation spectra and comparison with the experimental data. The table lists the energies of the ground state (GS) andnth excited states for QD helium and lithium, calculated using an exact diagonalization method (Etheo). Also shown are the leading configurations in the Slater determinant expansion with their relative contributions given in percent. Each level diagram represents an eigenstate to total spin and total angular momentum including the corresponding Slater determinants with permuted orbital configuration. For each degenerate spin and angular momentum multiplet, only one representative is shown. For QD helium, the good agreement betweenEtheoand the experimental valuesEexpmakes it possible to identify the GS and the first two excited states (triplet and singlet, respectively). The higher-lying resonances, seen in the fine structure of the QD helium spectrum, are also listed for comparison with the theoretically obtained values. Similarly, the theoretical and experimental values are listed for QD lithium. The experimentally determined values have an error of about 5% for QD helium and QD lithium. In Figure 4 , the calculated energies for the GS and the first few excited states are listed, together with the leading terms in the Slater determinant expansion (relative contributions given in %). Each level diagram represents an eigenstate to a total spin and total angular momentum including the corresponding Slater determinants with permuted orbital configuration. For each degenerate spin and angular momentum multiplet, only one representative is shown. Also shown are the experimental energies determined using the resonance condition for tunnelling E n − E n −1 =eΔ V p /λ and choosing the zero point of the energy scale such that the single-electron GS corresponds to E 1 GS = E (s1)=52 meV. Figure 4: Calculated excitation spectra and comparison with the experimental data. The table lists the energies of the ground state (GS) and n th excited states for QD helium and lithium, calculated using an exact diagonalization method ( E theo ). Also shown are the leading configurations in the Slater determinant expansion with their relative contributions given in percent. Each level diagram represents an eigenstate to total spin and total angular momentum including the corresponding Slater determinants with permuted orbital configuration. For each degenerate spin and angular momentum multiplet, only one representative is shown. For QD helium, the good agreement between E theo and the experimental values E exp makes it possible to identify the GS and the first two excited states (triplet and singlet, respectively). The higher-lying resonances, seen in the fine structure of the QD helium spectrum, are also listed for comparison with the theoretically obtained values. Similarly, the theoretical and experimental values are listed for QD lithium. The experimentally determined values have an error of about 5% for QD helium and QD lithium. Full size image Through a comparison between theory and experiment, we can clearly identify the double-peak structure in Figure 3a ( V p =−0.26 V and −0.2 V) as tunnelling into the triplet and singlet spin states of excited QD helium. The energy difference of about 10 meV is a direct measure of the exchange interaction in self-assembled QDs, which has so far only been studied in self-assembled dots using optical spectroscopy [9] , [5] . The splitting is large enough to allow for the all-electrical preparation of spin-polarized states. At a measuring time of 0.5 ms, about half of the addressed dots will be occupied (see the amplitude of the transient in Fig. 1c ). From a deconvolution of the double-peak structure, we can estimate that on the low-energy side of the resonance V p =−0.31 V, about 99% of the those dots will be prepared in the triplet state. The higher-lying resonances of QD helium are very closely spaced and therefore hardly discernible in the experiment. However, taking the calculations as a guide (see Fig. 4 ), they can be identified as tunnelling into different d-states of the dots; see also the comparison in Figure 4 . It should be pointed out that two of the corresponding calculated final states have an equally strong contribution from empty s-shells (see Fig. 4 , QD helium: third and sixth excited state). As the initial state is purely s-type, it is an interesting question how these contributions affect the tunnelling. However, to clarify the role of these contributions in the tunnelling process, a full calculation of the tunnelling dynamics, taking into account the Auger-type processes also would be necessary, which is beyond the scope of this work. The spectrum for QD lithium consists of a clear maximum at −0.16 V and a broad shoulder around +0.2 V. From comparison with theory and near equilibrium measurements [18] , we conclude that the low-energy resonance is caused by tunnelling into the three-electron GS. The additional resonances at higher energies are clear signatures of tunnelling into excited QD lithium states. Comparison with the calculated values in Figure 4 suggests that the observed fine structure corresponds to the first four excited QD lithium states. The measurement technique described here introduces the possibility to study time-resolved, non-equilibrium tunnelling phenomenon in self-assembled QD systems. This opens up a range of opportunities to investigate the structure and dynamics of excited states in these 'artificial atom-like' model systems. The observation of tunnelling into both singlet and triplet levels can be considered a first step towards an all-electrical manipulation and detection of spins in epitaxial QDs—a feat, which has so far only been possible in lithographically defined nanostructures [14] . Our findings also provide a link to the intriguing spin and interaction effects of self-assembled QDs, which have been identified using optical spectroscopy [26] . In conclusion, we have introduced a transport spectroscopic method that enables us to prepare and detect the many-particle spin states in self-assembled QDs by all-electrical means. The method introduced here for preparation and readout of quantum states in self-assembled structures has very favourable scaling properties: because the resistance of a 2D readout channel is only given by its length-to-width ratio, good signal-to-noise ratio is expected even for scaling down to the single-dot level—a prerequisite for quantum information technologies. To achieve single-dot addressing, a lateral spatial constriction of the 2DEG may be realized by etching [27] or by usage of split gates [28] . The random position of self-assembled QDs can be determined by atomic force microscopy, already demonstrated for positioning of a single QD inside a 2D photonic cavity [29] . To address many self-assembled QDs individually—a perquisite for quantum information processing—prepatterning techniques will have to be included to achieve a deterministic positioning of the dots [30] . Sample growth The sample is grown by solid-source molecular beam epitaxy on a GaAs(100) semi-insulating substrate. The active part of the structure starts with 150 nm Al 0.34 Ga 0.66 As, a Si-δ-doping, a 40 nm Al 0.34 Ga 0.66 and a spacer with the 2DEG at the interface. What follows is a tunnelling barrier of 15 nm GaAs, 10 nm Al 0.34 Ga 0.66 . As and 5 nm GaAs. On top of the GaAs layer, the InAs QDs are grown, followed by another 40 nm GaAs and an insulating AlAs/GaAs superlattice. Finally, the structure is capped with 5 nm GaAs. The dot density of the sample is about 8.3×10 9 cm −2 , determined by atomic force microscopic studies of similarly grown dots on the sample surface. Experimental setup The gated electron channel area is 5×10 3 μm 2 which leads to about 4×10 5 probed QDs. Hall measurements yield a charge carrier density and a mobility of the 2DEG of about 7.4×10 11 cm −2 and 9,340 cm 2 per V s , respectively. All measurements are performed in a He-cryostat at a temperature of 4.2 K, using a pulse generator at the gate contact and a current amplifier with a bandwidth of 1 MHz at the source contact. The drain contact is grounded and a bias of 30 mV is used at the current amplifier to measure the source-drain current I SD . How to cite this article: Marquardt, B. et al . Transport spectroscopy of non-equilibrium many-particle spin states in self-assembled quantum dots. Nat. Commun. 2:209 doi: 10.1038/1205 (2011).